Cytosolic p53 inhibits Parkin-mediated mitophagy and promotes mitochondrial dysfunction in the mouse heart Cumulative evidence indicates that mitochondrial dysfunction has a role in heart failure progression, but whether mitochondrial quality control mechanisms are involved in the development of cardiac dysfunction remains unclear. Here we show that cytosolic p53 impairs autophagic degradation of damaged mitochondria and facilitates mitochondrial dysfunction and heart failure in mice. Prevalence and induction of mitochondrial autophagy is attenuated by senescence or doxorubicin treatment in vitro and in vivo . We show that cytosolic p53 binds to Parkin and disturbs its translocation to damaged mitochondria and their subsequent clearance by mitophagy. p53-deficient mice show less decline of mitochondrial integrity and cardiac functional reserve with increasing age or after treatment with doxorubicin. Furthermore, overexpression of Parkin ameliorates the functional decline in aged hearts, and is accompanied by decreased senescence-associated β-galactosidase activity and proinflammatory phenotypes. Thus, p53-mediated inhibition of mitophagy modulates cardiac dysfunction, raising the possibility that therapeutic activation of mitophagy by inhibiting cytosolic p53 may ameliorate heart failure and symptoms of cardiac ageing. Heart failure is a complex pathophysiological syndrome that arises from a primary defect in the pumping capacity of the heart to match the body’s demands [1] . There are many reasons why a human heart can fail, but the available evidence suggests that a functional decline of mitochondria is one of the major mechanisms underlying heart failure progression [2] , [3] , [4] . Impaired mitochondria provoke energy-generation defects, the increased production of harmful reactive oxygen species (ROS), and a greater propensity to trigger apoptosis [5] . Cardiac myocytes are abundant in mitochondria for their high-energy demands and as a result, are particularly vulnerable to mitochondrial compromise. Recent evidence has revealed that mitochondrial integrity is maintained by the dynamic nature of the mitochondrial population in the cell. Membrane fusion and fission allow mitochondrial content mixing within a cell to maintain integrity, and severely damaged mitochondria are selectively removed by macroautophagy, termed mitophagy [6] , [7] , [8] . PINK1 and Parkin have been shown to have important roles in the induction of mitophagy [9] , [10] . PINK1 is imported into healthy mitochondria and rapidly degraded by proteolysis, and is then maintained at very low levels. When mitochondria are damaged and lose membrane potential, PINK1 accumulates and recruits the E3 ubiquitin ligase Parkin, leading to the ubiquitination of mitochondrial substrates including the outer membrane protein VDAC1 (ref. 11 ), Mfn1 and Mfn2 (ref. 12 ). This modification recruits the autophagy adaptor molecule, p62/SQSTM1, and thereby targets mitochondria for autophagic removal [11] . Moreover, the proteasomal degradation of MFN1 and MFN2 inhibits mitochondrial fusion and facilitates mitophagy [12] . The efficient removal of dysfunctional mitochondria is crucial to maintain cellular homeostasis in tissues comprised of non-dividing cells because damaged organelles cannot be diluted by cell proliferation [13] . Ageing is a major risk factor for heart failure and mitochondrial dysfunction is also central to theories of ageing. Mitochondrial function and mitochondrial DNA (mtDNA) quality were shown to decline with age in postmitotic tissues [14] , [15] , [16] , [17] , and several recent studies, reporting on defects in mtDNA quality control mechanisms in mice, have shown that these mutant animals develop a phenotype of premature aging [17] , [18] . Given these findings, mitochondrial quality control may be associated with aging-related decreases in cardiac contractility and the pathogenesis of specific heart diseases that are especially caused by mitochondrial dysfunction including doxorubicin (DOX)-induced cardiotoxicity [19] . In the present study, we investigated the impact of Parkin-mediated mitophagy on cardiac aging and DOX cardiotoxicity. We found a novel protein–protein interaction between the p53 tumour suppressor protein and Parkin in cytosol. The inhibitory action of p53 on Parkin-mediated mitophagy exacerbates mitochondrial compromise and heart failure in addition to classical cell fate decisions concerning senescence or apoptosis. Mitochondrial autophagy in aged and DOX-treated hearts To highlight the impact of mitochondrial quality control on the process of aging, we evaluated mitochondrial autophagy in hearts that were or were not treated with the mitochondrial uncoupler, carbonyl cyanide p -trichloromethoxyphenylhydrazone (CCCP). Hearts were collected 12 h after an intraperitoneal injection of 5 mg kg −1 CCCP. Electron microscopy revealed that mitochondria incorporated into autophagic vacuoles were found more in the hearts of adult (10-month old) mice under both baseline and CCCP-treated conditions ( Fig. 1a ) than in the hearts of aged (20-month old) mice. Immunohistochemistry of GFP-LC3 transgenic mice hearts also demonstrated that colocalization between a marker of autophagosomes, LC3, and mitochondria was decreased in aged mice ( Supplementary Fig. S1 ). In the fractionation experiment, the expression of Parkin and PINK1 did not differ with age, whereas CCCP-induced Parkin translocation from cytosol to mitochondria and subsequent recruitment of p62 were attenuated in the hearts of aged mice ( Fig. 1b ). We then administered DOX in five equal intraperitoneal injections over a period of 2 weeks with a total cumulative dosage of 12.5 mg kg −1 at 10 weeks of age ( Supplementary Fig. S2a ) to examine DOX cardiomyopathy, the pathogenesis of which was shown to be mainly affected by mitochondrial dysfunction [19] . In addition, DOX-treated hearts exhibited aging-related alterations including the upregulation of SA-β-gal activity and expression of cell cycle inhibitors and proinflammatory cytokines ( Supplementary Fig. S2b–d ) [20] , [21] , [22] . CCCP-induced Parkin and p62 translocation was also reduced in DOX-treated hearts ( Fig. 1c ). 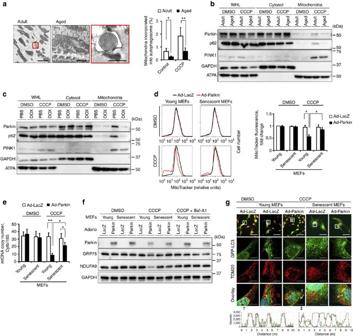Figure 1: Mitophagy is impaired in aged and DOX-treated hearts. (a) Ten-month-old adult mice and 20-month-old aged mice were treated with an intraperitoneal injection of 5 mg kg−1CCCP and their hearts were collected 12 h later. Representative electron micrographs of hearts from CCCP-treated adult and aged mice; original magnification × 5,000; scale bar, 2 μm. The magnified photograph represents an autophagic vacuole containing mitochondria; original magnification × 12,000; scale bar, 500 nm. Mitochondria incorporated into an autophagic vacuole in baseline and CCCP-treated conditions were quantified blindly from 8–10 images from different fields (original magnification × 5,000) (n=3 per group). (b,c) CCCP-induced recruitment of Parkin and p62 to mitochondria was determined by immunoblotting of the heart mitochondria-rich fraction in adult and aged mice (b), and DOX-treated mice (c). Representative immunoblots are shown from four independent experiments. (d) Parkin was overexpressed in young and senescent MEFs using adenovirus-mediated transduction for thein vitrocell-based bioassay to assess the ability to clear damaged mitochondria. Mitochondrial content after 24 h of treatment with 20 μM CCCP was assessed by flow cytometry for MitoTracker Green FM. Results from four independent experiments performed in duplicate are shown. MEFs at passage 3 and passage 9 were used as young and senescent MEFs, respectively. (e) Mitochondrial DNA content was assessed by real-time PCR. Results are shown from six-independent experiments. (f) Mitochondrial content was assessed by immunoblotting for the mitochondrial chaperone, GRP75 (matrix protein) and complex I subunit, NDUFA9 (inner membrane protein). MEFs were treated with 100 nM bafilomycin-A1, (Baf-A1, an inhibitor of the vacuolar-type proton ATPase) to inhibit autophagy. Representative immunoblots are shown from three independent experiments. (g) Representative images of GFP-LC3 expressing MEFs treated with 20 μM CCCP for 10 h before the immunostaining of mitochondria with anti-TOM20 (red); original magnification, × 400 and × 1,000; scale bar, 100 μm and scale bar, 15 μm. Line scans below the images indicate colocalization between LC3 (green) and mitochondria (red) and correlate to the arrows drawn in the images. WHL indicates whole-heart lysate. Data are shown as the means±s.d. *P<0.05; **P<0.01 (two-tailed unpaired Student’st-test). Figure 1: Mitophagy is impaired in aged and DOX-treated hearts. ( a ) Ten-month-old adult mice and 20-month-old aged mice were treated with an intraperitoneal injection of 5 mg kg −1 CCCP and their hearts were collected 12 h later. Representative electron micrographs of hearts from CCCP-treated adult and aged mice; original magnification × 5,000; scale bar, 2 μm. The magnified photograph represents an autophagic vacuole containing mitochondria; original magnification × 12,000; scale bar, 500 nm. Mitochondria incorporated into an autophagic vacuole in baseline and CCCP-treated conditions were quantified blindly from 8–10 images from different fields (original magnification × 5,000) ( n =3 per group). ( b , c ) CCCP-induced recruitment of Parkin and p62 to mitochondria was determined by immunoblotting of the heart mitochondria-rich fraction in adult and aged mice ( b ), and DOX-treated mice ( c ). Representative immunoblots are shown from four independent experiments. ( d ) Parkin was overexpressed in young and senescent MEFs using adenovirus-mediated transduction for the in vitro cell-based bioassay to assess the ability to clear damaged mitochondria. Mitochondrial content after 24 h of treatment with 20 μM CCCP was assessed by flow cytometry for MitoTracker Green FM. Results from four independent experiments performed in duplicate are shown. MEFs at passage 3 and passage 9 were used as young and senescent MEFs, respectively. ( e ) Mitochondrial DNA content was assessed by real-time PCR. Results are shown from six-independent experiments. ( f ) Mitochondrial content was assessed by immunoblotting for the mitochondrial chaperone, GRP75 (matrix protein) and complex I subunit, NDUFA9 (inner membrane protein). MEFs were treated with 100 nM bafilomycin-A1, (Baf-A1, an inhibitor of the vacuolar-type proton ATPase) to inhibit autophagy. Representative immunoblots are shown from three independent experiments. ( g ) Representative images of GFP-LC3 expressing MEFs treated with 20 μM CCCP for 10 h before the immunostaining of mitochondria with anti-TOM20 (red); original magnification, × 400 and × 1,000; scale bar, 100 μm and scale bar, 15 μm. Line scans below the images indicate colocalization between LC3 (green) and mitochondria (red) and correlate to the arrows drawn in the images. WHL indicates whole-heart lysate. Data are shown as the means±s.d. * P <0.05; ** P <0.01 (two-tailed unpaired Student’s t -test). Full size image Parkin-mediated mitophagy is attenuated in senescent MEFs Next, we examined the effect of cellular senescence on the induction of mitophagy. For in vitro cell-based bioassay to assess the ability to clear impaired mitochondria, we expressed Parkin using adenovirus-mediated transduction in mouse embryo fibroblasts (MEFs) and treated with 20 μM CCCP for 24 h. Mitochondrial content was assessed by using flow cytometry for MitoTracker Green FM that fluoresces independently of mitochondrial [Ca 2+ ] and membrane potential, real-time PCR to quantify mtDNA content, and immunoblotting for GRP75 (mitochondrial chaperone, matrix protein) and NDUFA9 (complex I subunit, inner membrane protein). CCCP-induced mitochondrial clearance was markedly lower in senescent MEFs than in young MEFs ( Fig. 1d–f ). To demonstrate that mitochondria were actually degraded by an autophagic process, we confirmed that inhibiting autophagy with bafilomycin-A1 (Baf-A1) or 3-methyladenine cancelled mitochondrial clearance ( Fig. 1f and Supplementary Fig. S3 ). We also assessed colocalization between LC3 and mitochondria after mitochondrial depolarization using MEFs infected with adenovirus GFP-LC3. Colocalization between fragmented mitochondria and LC3-labelled autophagosomes was seen in Parkin expressing young MEFs after 10 h of the CCCP treatment ( Fig. 1g ). p53 is involved in the defect of Parkin-mediated mitophagy Senescence-inducing signal transductions have two major pathways: one is mediated by p53 and p21, a cyclin-dependent kinase inhibitor and the other by p16, another cyclin-dependent kinase inhibitor. Retinoblastoma protein (Rb) is a downstream target of both. Oncogenic RAS engages both pathways to induce premature senescence [23] . To test the contribution to mitophagy deficiency in senescent cells, we overexpressed these molecules in MEFs using retroviral-mediated gene transfer. p53 and H-Ras 12V overexpression in MEFs was accompanied by the impairment of mitophagy. In contrast, p53-downstream or p53-independent mediators, p21, p16 and Rb had no significant effects on mitophagy ( Fig. 2a ). Moreover, mitochondrial clearance was preserved against the H-Ras 12V transgene in p53 −/− MEFs, not in p21 −/− MEFs ( Fig. 2c ). The knockdown of p53 with a specific short interfering (si) RNA or pifithrin-α recovered mitochondrial clearance in H-Ras 12V expressing wild-type (WT) MEFs, but did not affect any further decreases in p53 −/− MEFs ( Fig. 2d ). In addition to confirming the autophagic process ( Fig. 2b ), we discriminated the effect of mitochondrial biogenesis on the decrease of mitochondrial content. Peroxisome proliferator-activated receptor gamma coactivator (PGC)-1α expression was obviously enhanced in association with mitochondrial reduction, which was thought to be a compensative response to maintain mitochondrial content ( Supplementary Fig. S4a ). These results suggested that p53 was responsible for the impaired Parkin-mediated mitophagy in senescent MEFs. We also performed experiments using the murine HL-1 cardiac myocyte cell line, in which Parkin overexpression did not affect the expression of PGC-1α and p53 ( Supplementary Fig. S4b ). Retrovirus-mediated p53 transduction disturbed Parkin-mediated mitophagy in HL-1 cells ( Fig. 2e ). The levels of expression achieved by retroviral gene transfer did not exceed endogenous levels of expression in MEFs and HL-1 cells ( Supplementary Fig. S4c ). siRNA targeting p53, not p21 and p16, preserved mitochondrial clearance under the low concentration of 0.02 μM DOX treatment in HL-1 cells ( Supplementary Fig. S4d , Fig. 2f ), which induced senescence-like phenotypes including higher SA-β-gal activity and expressions of cell cycle inhibitors [20] ( Supplementary Figs S4c,S5a,b ). In DOX-treated hearts, CCCP-mediated Parkin translocation and the subsequent biological response including the degradation of Mfn1 (ref. 12 ) were preserved in p53 −/− hearts without any alterations of other mitochondrial dynamics associated proteins such as Drp1. p21 −/− hearts revealed no alterations in protein dynamics ( Fig. 2g ). Parkin-mediated mitophagy deficiency with p53 involvement in senescent MEFs was also observed in HL-1 cells and hearts exposed to DOX toxicity. 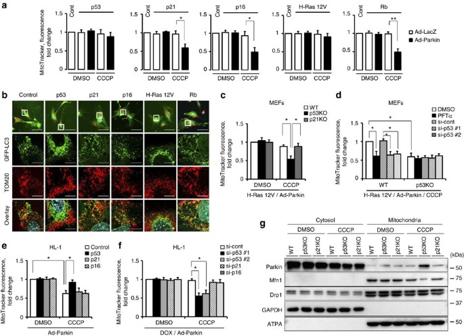Figure 2: p53 contributes to Parkin-mediated mitophagy deficiency. (a) The senescence-associated molecules p53, p21, p16, H-Ras 12V and Rb were overexpressed in MEFs by retrovirus-mediated transduction. After puromycin selection, mitophagy induction was performed with treatment of 20 μM CCCP 24 h after adenovirus-mediated Parkin expression. Mitochondrial content 24 h after mitophagy induction was assessed by flow cytometry for MitoTracker Green FM. Results are shown from four independent experiments performed in duplicate. (b) Representative images of MEFs infected with the GFP-LC3 adenovirus and stained with anti-TOM20 (red) to visualize mitochondria 10 h after mitophagy induction; original magnification, × 400 and × 1,000; scale bar, 100 μm and scale bar, 15 μm. (c) Mitochondrial content of H-Ras 12 V expressing WT,p53−/−andp21−/−MEFs was assessed by flow cytometry 24 h after mitophagy induction. Results are shown from four independent experiments performed in duplicate. (d) Mitochondrial content of WT andp53−/−MEFs was assessed by flow cytometry 24 h after mitophagy induction. WT andp53−/−MEFs were transfected with control or p53-specific siRNAs or cultured in complete medium for 24 h in the presence or absence of 20 μM pifithrin-α before mitophagy induction. Results are shown from four independent experiments performed in duplicate. (e) Murine HL-1 cardiac myocytes were infected with retrovirus vectors encoding p53, p21 or p16 and after puromycin selection, underwent mitophagy induction. Mitochondrial content is assessed by flow cytometry from four independent experiments performed in duplicate are shown. (f) HL-1 cells were transfected with control, p53, p21 or p16-specific siRNAs, followed by treatment with 0.02 μM DOX and mitophagy induction. Mitochondrial content is assessed by flow cytometry from four independent experiments performed in duplicate. (g) CCCP-induced recruitment of Parkin and expression of Mfn1 and Drp1 in DOX-treated WT,p53−/−andp21−/−mice were determined by immunoblotting of the heart mitochondria-rich fraction. Representative immunoblots are shown from four independent experiments. Data are shown as the means±s.d. *P<0.05; **P<0.01 (two-tailed unpaired Student’st-test). Figure 2: p53 contributes to Parkin-mediated mitophagy deficiency. ( a ) The senescence-associated molecules p53, p21, p16, H-Ras 12V and Rb were overexpressed in MEFs by retrovirus-mediated transduction. After puromycin selection, mitophagy induction was performed with treatment of 20 μM CCCP 24 h after adenovirus-mediated Parkin expression. Mitochondrial content 24 h after mitophagy induction was assessed by flow cytometry for MitoTracker Green FM. Results are shown from four independent experiments performed in duplicate. ( b ) Representative images of MEFs infected with the GFP-LC3 adenovirus and stained with anti-TOM20 (red) to visualize mitochondria 10 h after mitophagy induction; original magnification, × 400 and × 1,000; scale bar, 100 μm and scale bar, 15 μm. ( c ) Mitochondrial content of H-Ras 12 V expressing WT, p53 −/− and p21 −/− MEFs was assessed by flow cytometry 24 h after mitophagy induction. Results are shown from four independent experiments performed in duplicate. ( d ) Mitochondrial content of WT and p53 −/− MEFs was assessed by flow cytometry 24 h after mitophagy induction. WT and p53 −/− MEFs were transfected with control or p53-specific siRNAs or cultured in complete medium for 24 h in the presence or absence of 20 μM pifithrin-α before mitophagy induction. Results are shown from four independent experiments performed in duplicate. ( e ) Murine HL-1 cardiac myocytes were infected with retrovirus vectors encoding p53, p21 or p16 and after puromycin selection, underwent mitophagy induction. Mitochondrial content is assessed by flow cytometry from four independent experiments performed in duplicate are shown. ( f ) HL-1 cells were transfected with control, p53, p21 or p16-specific siRNAs, followed by treatment with 0.02 μM DOX and mitophagy induction. Mitochondrial content is assessed by flow cytometry from four independent experiments performed in duplicate. ( g ) CCCP-induced recruitment of Parkin and expression of Mfn1 and Drp1 in DOX-treated WT, p53 −/− and p21 −/− mice were determined by immunoblotting of the heart mitochondria-rich fraction. Representative immunoblots are shown from four independent experiments. Data are shown as the means±s.d. * P <0.05; ** P <0.01 (two-tailed unpaired Student’s t -test). Full size image Cytosolic p53 binds to the RING0 domain of Parkin The reduced expression of molecules associated with mitochondrial quality control and biogenesis were not observed in aged hearts ( Supplementary Fig. S6a ). To elucidate mechanisms underlying the mitophagy deficiency in aging, we searched for the protein interacting with p53 using an epitope-tagged protein in HL-1 cells. An apparent protein–protein interaction between p53 and Parkin was observed under DOX treatment ( Fig. 3a ) which had no effect on Parkin expression at the transcriptional level ( Supplementary Fig. S6b ). The interaction of endogenous proteins was detected in rat neonatal cardiomyocytes under the H 2 O 2 as treatment well as DOX, and it became prominent in parallel with p53 expression ( Fig. 3b ). Analysis of two-step immunoprecipitation with the cytosolic lysate of the heart [24] revealed that this interaction was enhanced in aged mice with an apparent upregulation of cytosolic p53 expression ( Supplementary Fig. S7a,b ). We also confirmed the endogenous Parkin–p53 complex in both immunoprecipitates of endogenous Parkin and p53 prominently in the cytosolic lysate of aged hearts ( Fig. 3c ). We next investigated the domain-structure of Parkin to determine the region that contributes to the interaction with p53. Parkin is divided into three parts: the N-terminal Ubl domain, the C-terminal RING-box and the RING0 region. The C-terminal RING box region consists of three domains termed RING1, RING2 and IBR (for in-between-RING) ( Fig. 3d ) [25] . Various FLAG-tagged human Parkin mutants were transfected to DOX-treated HeLa cells. An immunoprecipitation assay revealed that the RING0 domain was essential to interact with p53, because deletion of the Ubl domain had no effect on binding, and RING box alone caused a loss in the ability to bind to p53 ( Fig. 3e ). To reveal the region of p53 that is responsible for the interaction, we further performed GST pull-down assays using GST–p53 fusion proteins ( Fig. 3f ). Residues 81–160 of p53 were sufficient to mediate the Parkin interaction ( Fig. 3g ). 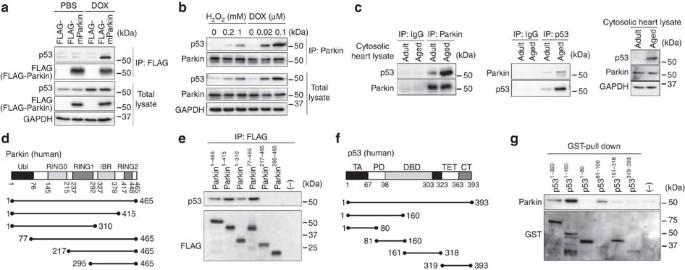Figure 3: Protein interaction of p53 with Parkin and domain analysis. (a) Whole-cell lysates of HL-1 cells treated with 0.02 μM DOX and transfected with FLAG-tagged Parkin or the FLAG-empty vector were immunoprecipitated with the anti-Flag-M2 antibody and blotted with anti-p53 and Flag antibodies. (b) Whole-cell lysates of rat neonatal cardiomyocytes treated with the indicated concentrations of H2O2and DOX for 24 h were immunoprecipitated with the anti-Parkin antibody. (c) Cytosolic heart lysates of adult and aged mice were immunoprecipitated with anti-Parkin, p53 and control IgG antibodies. (d) Schematic representation of N-terminally FLAG-tagged WT Parkin and various mutants of Parkin. (e) The association of endogenous p53 with various Parkin mutants in DOX-treated HeLa cells. The immunoprecipitation assay revealed that the RING0 domain was essential for the interaction with p53. (f) Schematic representation of the GST–p53 fusion proteins. (g) GST pull-down assays using GST–p53 fusion proteins andin vitrotranscribed/translated FLAG-Parkin. Residues 81–160 of p53 were sufficient to bind Parkin. Figure 3: Protein interaction of p53 with Parkin and domain analysis. ( a ) Whole-cell lysates of HL-1 cells treated with 0.02 μM DOX and transfected with FLAG-tagged Parkin or the FLAG-empty vector were immunoprecipitated with the anti-Flag-M2 antibody and blotted with anti-p53 and Flag antibodies. ( b ) Whole-cell lysates of rat neonatal cardiomyocytes treated with the indicated concentrations of H 2 O 2 and DOX for 24 h were immunoprecipitated with the anti-Parkin antibody. ( c ) Cytosolic heart lysates of adult and aged mice were immunoprecipitated with anti-Parkin, p53 and control IgG antibodies. ( d ) Schematic representation of N-terminally FLAG-tagged WT Parkin and various mutants of Parkin. ( e ) The association of endogenous p53 with various Parkin mutants in DOX-treated HeLa cells. The immunoprecipitation assay revealed that the RING0 domain was essential for the interaction with p53. ( f ) Schematic representation of the GST–p53 fusion proteins. ( g ) GST pull-down assays using GST–p53 fusion proteins and in vitro transcribed/translated FLAG-Parkin. Residues 81–160 of p53 were sufficient to bind Parkin. Full size image p53 inhibits Parkin translocation to mitochondria We confirmed the contribution of p53 to Parkin-mediated mitophagy in GFP-mParkin overexpressing HL-1 cells, which showed signs of mitochondrial translocation, sequestration and clearance with the CCCP treatment. Prior treatment with DOX significantly attenuated Parkin recruitment to mitochondria and subsequent mitochondrial ubiquitination 6 h after the CCCP treatment as well as mitochondrial clearance within 24 h. Nutlin-3, a nongenotoxic activator of the p53 pathway, had similar effects on the dynamics of Parkin, whereas the knockdown of p53 with siRNA restored Parkin translocation and clearance. A similar analysis with siRNAs targeting p16 and p21 revealed no alterations in Parkin localization ( Supplementary Fig. S8a–f ). We confirmed the redistribution of endogenous Parkin and subsequent ubiquitination of mitochondria proteins such as VDAC1 (ref. 11 ) using fractionation experiments and immunoprecipitation in HL-1 cells ( Fig. 4a , Supplementary Fig. S9a,b ). The protein interaction and the inhibitory effect on Parkin-mediated mitophagy were observed in parallel with p53 expression in DOX-treated YFP-Parkin expressing HCT116 cells ( Supplementary Fig. S10a–f ). We also determined that cytosolic, not nuclear, p53 inhibited Parkin-mediated mitophagy using YFP-Parkin expressing p53 −/− HCT116 cells re-transfected with p53 targeted to nuclear or extra-nuclear location ( Supplementary Fig. S11a ). The levels of protein expression achieved did not exceed that of biological expression ( Supplementary Fig. S11b ). WT p53 inhibited Parkin translocation and subsequent mitophagy, whereas a p53 form locked into the nucleus (using a disrupted nuclear export signal, NES) and an endoplasmic reticulum (ER)-targeted p53 (p53 ER) failed to inhibit the process of mitophagy. A p53 mutant with a mutation in the NLS (nuclear localization sequence), which causes cytosolic retention of p53, efficiently inhibited mitophagy. The N-terminally truncated isoforms Δ40p53 and Δ133p53 were also re-transfected. Mitophagy was disturbed by Δ40p53, not Δ133p53, consistent with the results of the domain analysis ( Fig. 4c–g ). 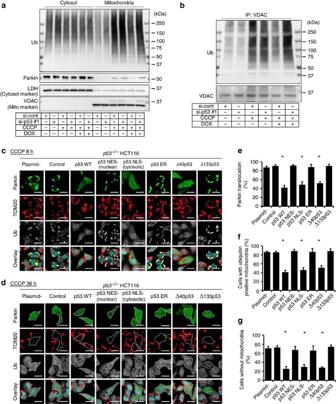Figure 4: Cytosolic p53 interrupts the mitochondrial translocation of Parkin. (a) HL-1 cells transfected with control or p53-specific siRNAs no.1 and cultured in complete medium for 24 h in the presence or absence of 0.02 μM DOX. After treatment with 20 μM CCCP for 6 h, the fractionation experiment was performed. Endogenous Parkin translocation to mitochondria and ubiquitination were assessed by immunoblotting. Representative immunoblots are shown from three independent experiments. (b) These samples were subjected to immunoprecipitation with the anti-VDAC antibody to evaluate ubiquitination. Representative immunoblots are shown from three independent experiments. (c,d) Representative images of YFP-Parkin overexpressingp53−/−HCT116 cells re-transfected with WT p53 and various mutants of p53 and treated with 60 μM CCCP for 8 (c) and 36 h (d) before the immunostaining of mitochondria with anti-TOM20 (red) and endogenous poly-ubiquitin with a specific antibody FK-2 (white); original magnification, × 630; scale bar, 20 μm. (e–g) Parkin mitochondrial translocation (e) and ubiquitination (f) 8 h after CCCP treatment and mitochondrial clearance (g) 36 h after CCCP treatment were quantified. A minimum of 300–400 YFP-positive cells were scored in three independent experiments. The single-letter amino-acid code is used. NES indicates nuclear export signal; NLS, nuclear localization signal; ER, endoplasmic reticulum; Ub, ubiquitin. Data are shown as the means±s.d. *P<0.05, compared with the corresponding control (two-tailed unpaired Student’st-test). Figure 4: Cytosolic p53 interrupts the mitochondrial translocation of Parkin. ( a ) HL-1 cells transfected with control or p53-specific siRNAs no.1 and cultured in complete medium for 24 h in the presence or absence of 0.02 μM DOX. After treatment with 20 μM CCCP for 6 h, the fractionation experiment was performed. Endogenous Parkin translocation to mitochondria and ubiquitination were assessed by immunoblotting. Representative immunoblots are shown from three independent experiments. ( b ) These samples were subjected to immunoprecipitation with the anti-VDAC antibody to evaluate ubiquitination. Representative immunoblots are shown from three independent experiments. ( c , d ) Representative images of YFP-Parkin overexpressing p53 −/− HCT116 cells re-transfected with WT p53 and various mutants of p53 and treated with 60 μM CCCP for 8 ( c ) and 36 h ( d ) before the immunostaining of mitochondria with anti-TOM20 (red) and endogenous poly-ubiquitin with a specific antibody FK-2 (white); original magnification, × 630; scale bar, 20 μm. ( e–g ) Parkin mitochondrial translocation ( e ) and ubiquitination ( f ) 8 h after CCCP treatment and mitochondrial clearance ( g ) 36 h after CCCP treatment were quantified. A minimum of 300–400 YFP-positive cells were scored in three independent experiments. The single-letter amino-acid code is used. NES indicates nuclear export signal; NLS, nuclear localization signal; ER, endoplasmic reticulum; Ub, ubiquitin. Data are shown as the means±s.d. * P <0.05, compared with the corresponding control (two-tailed unpaired Student’s t -test). Full size image p53 attenuates mitophagy and promotes DOX cardiotoxicity We evaluated the effects of the inhibitory interaction of p53 with Parkin on mitochondrial biology in DOX cardiotoxicity. DOX-treated p53 −/− mice had more mitochondria incorporated into autophagosomes ( Fig. 5a ), which inversely correlated with abnormal mitochondrial structure ( Fig. 5c ) and oxidative stress in mtDNA ( Fig. 5d ). Parkin −/− mice exhibited less mitochondrial autophagy and more impaired mitochondrial integrity, which was not salvaged by p53 depletion. p21 −/− mice did not show any protective effect on mitochondrial quality unlike p53 −/− mice ( Fig. 5a–d ). The functional compromise of mitochondria was substantiated by respiration studies of isolated heart mitochondria. A sequential state III respiration assay revealed that DOX-treated hearts were significantly reduced in complexes I-, II-, IV-driven O 2 consumption in WT, which was ameliorated in p53 −/− mice. Parkin −/− mice exhibited the advanced respiratory compromise and p53 −/− Parkin −/− mice failed to mitigate mitochondrial damage ( Supplementary Fig. S12a,b ). This impaired mitochondrial respiration paralleled a reduction in ATP content in dobutamine-loaded hearts ( Supplementary Fig. S12c ). Cardiac functional reserve assessed by the response of maximum dP/dt using cardiac catheterization under dobutamine loading reflected this energy compromise ( Fig. 5e ). In PBS-treated control hearts, reduced complex IV-driven O 2 consumption and energy compromise under dobutamine loading were seen in p53 −/− mice ( Supplementary Fig. S12a–c ), consistent with previous reports showing that p53 was associated with mitochondrial function and complex IV activity through SCO2 (ref. 26 ). 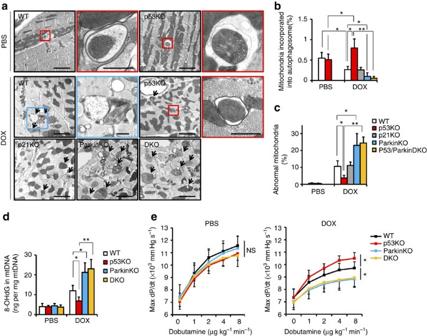Figure 5: Interaction of p53 with Parkin contributes to DOX-induced cardiotoxicity. (a) Representative electron micrographs of DOX-treated hearts. Arrows indicate abnormal mitochondria defined by marked swelling, vacuolation (loss of electron density) or disrupted cristae; original magnification × 5,000; scale bar, 2 μm. The magnified photograph represents abnormal mitochondria (blue line) and an autophagic vacuole containing mitochondria (red line); original magnification × 12,000; scale bar, 500 nm. (b,c) Mitochondria incorporated into an autophagic vacuole (b) and abnormal mitochondria (c) were quantified blindly from 8–10 images from different fields (original magnification × 5,000) (n=3 per group). (d) The 8-hydroxy-2′-deoxyguanosine (8-OHdG), popular marker for oxidative DNA damage, in mitochondria DNA from DOX-treated hearts. Results are shown from 6–8 hearts analysed in duplicate. (e) Maximum dP/dt was examined using cardiac catheterization under graded dobutamine infusion in PBS-treated (control) and DOX-treated mice (n=6–8 per group). DKO indicates double knockout. Data are shown as the means±s.d. *P<0.05; **P<0.01 (two-tailed unpaired Student’st-test). Figure 5: Interaction of p53 with Parkin contributes to DOX-induced cardiotoxicity. ( a ) Representative electron micrographs of DOX-treated hearts. Arrows indicate abnormal mitochondria defined by marked swelling, vacuolation (loss of electron density) or disrupted cristae; original magnification × 5,000; scale bar, 2 μm. The magnified photograph represents abnormal mitochondria (blue line) and an autophagic vacuole containing mitochondria (red line); original magnification × 12,000; scale bar, 500 nm. ( b , c ) Mitochondria incorporated into an autophagic vacuole ( b ) and abnormal mitochondria ( c ) were quantified blindly from 8–10 images from different fields (original magnification × 5,000) ( n =3 per group). ( d ) The 8-hydroxy-2′-deoxyguanosine (8-OHdG), popular marker for oxidative DNA damage, in mitochondria DNA from DOX-treated hearts. Results are shown from 6–8 hearts analysed in duplicate. ( e ) Maximum dP/dt was examined using cardiac catheterization under graded dobutamine infusion in PBS-treated (control) and DOX-treated mice ( n =6–8 per group). DKO indicates double knockout. Data are shown as the means±s.d. * P <0.05; ** P <0.01 (two-tailed unpaired Student’s t -test). Full size image p53 and mitochondrial integrity in cardiac aging To evaluate the role of Parkin-mediated mitophagy in cardiac aging, we examined the age-dependent decline of mitochondrial integrity and cardiac function across a wide range of ages in Parkin −/− mice. The age-dependent accumulation of mtDNA deletion mutations and oxidative damage was promoted in Parkin −/− mice ( Supplementary Fig. S13a,b ). The functional decline of mitochondrial respiration assessed by complex I dependent state III O 2 consumption and the ATP synthesis rate was also accelerated in Parkin − /− mice ( Supplementary Fig. S13c,d ). These underlay the decline of cardiac functional reserve assessed by the response of maximal and minimal dP/dt against dobutamine infusion ( Supplementary Fig. S13e ). Moreover, the hearts of 15-month-old Parkin −/− mice showed enhanced SA-β-gal activity ( Supplementary Fig. S13f ). The reduced life spans of Parkin −/− mice have also been previously reported [27] . Given evidence of accelerated aging phenotype in Parkin −/− mice indicates that the maintenance of mitochondrial integrity and healthy aging requires Parkin-mediated mitochondrial quality control. Based on these results, we investigated the influence of a p53-mediated mitophagy deficiency on cardiac aging, using 20-month-old heterozygous littermates surviving grossly tumour free; 92% of WT (48 out of 52), 28% of p53 +/− (14 out of 50), 94% of Parkin +/− (45 out of 48) and 21% of p53 +/− Parkin +/− (10 out of 48). The sequential state III respiration assay revealed that complexes I-, II-, IV-driven O 2 consumption in the aged heart was significantly higher in p53 +/− littermates than in the other littermates ( Fig. 6a ). Age-dependent declines of mitochondrial membrane potential and particle size enlargements assessed by flow cytometry of isolated mitochondria were also mitigated in aged p53 +/− littermates ( Fig. 6c ). ROS generation when NADH was used as the complex I-linked substrate was also ameliorated in aged p53 +/− littermates, whereas maximally stimulated ROS generation from complex I in the presence of rotenone was marked, reflecting the preserved enzymatic activity of the respiratory complex ( Fig. 6e ). Preserved mitochondrial integrity resulted in improved myocardial high-energy phosphate metabolism in dobutamine-loaded hearts ( Fig. 6f ). Cardiac functional reserve was maintained in p53 +/− aged littermates in correlation with energy homeostasis ( Fig. 6g ). SA-β-gal activity was reduced in p53 +/− aged littermates, which was dependent on Parkin. The p53-mediated interruption of mitophagy contributed to not only the functional decline but aging biomarker expression ( Fig. 6h ). 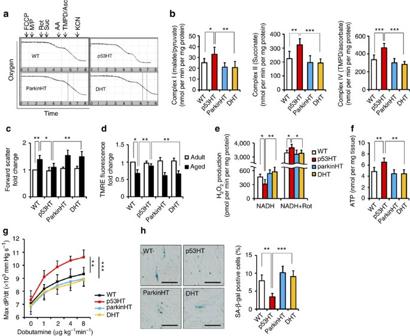Figure 6: p53-mediated mitophagy deficiency and biological cardiac aging. We used 20-month-old heterozygous littermates surviving grossly tumor free. (a,b) The sequential state III oxygen consumption rate of heart isolated mitochondria (300 μg) was monitored with a fibre-optic system. Substrates and inhibitors were added sequentially at the final concentrations indicated as follow. FCCP, 1 μM carbonylcyanide-p-trifluoromethoxyphenylhydrazone; M/P, 5 mM malate+5 mM pyruvate; Rot, 100 nM rotenone; Suc, 5 mM succinate; AA, 50 nM antimycin A; TMPD/Asc, 0.4 mM N,N,N′,N′-tetramethyl-p-phenylenediamine +1 mM ascorbate; KCN, 5 mM potassium cyanide. Representative results are shown (a) and oxygen consumption by each complex was calculated (n=5–8 per group,b). (c,d) Mitochondrial particle size (c) and membrane potential (d) were determined using flow cytometry for TMRE in cardiac mitochondria preparations. Results are shown from 4–8 hearts analysed in duplicate. (e) H2O2production with 0.5 mM NADH, complex I-linked substrate, was determined in the absence or presence of 2 μM complex I inhibitor rotenone using Amplex Red (n=5–8 per group). (f) Myocardial high-energy phosphate metabolism under 8γ dobutamine loading was measured biochemically with HPLC (n=5 per group). (g) Maximum dP/dt was examined using cardiac catheterization with graded a dobutamine infusion (n=5 per group). (h) Photographs showing heart sections after SA-β-gal staining; original magnification, × 200; scale bar, 40 μm. SA-β-gal-positive cells were quantified (n=4 per group). Five images per mouse were taken on brightfield and DAPI staining was used to count the total cell number per section. HT indicates heterozygous; DHT double heterozygous. Data are shown as the means±s.d. *P<0.05; **P<0.01; ***P<0.001 (two-tailed unpaired Student’st-test). Figure 6: p53-mediated mitophagy deficiency and biological cardiac aging. We used 20-month-old heterozygous littermates surviving grossly tumor free. ( a , b ) The sequential state III oxygen consumption rate of heart isolated mitochondria (300 μg) was monitored with a fibre-optic system. Substrates and inhibitors were added sequentially at the final concentrations indicated as follow. FCCP, 1 μM carbonylcyanide-p-trifluoromethoxyphenylhydrazone; M/P, 5 mM malate+5 mM pyruvate; Rot, 100 nM rotenone; Suc, 5 mM succinate; AA, 50 nM antimycin A; TMPD/Asc, 0.4 mM N,N,N′,N′-tetramethyl- p -phenylenediamine +1 mM ascorbate; KCN, 5 mM potassium cyanide. Representative results are shown ( a ) and oxygen consumption by each complex was calculated ( n =5–8 per group, b ). ( c , d ) Mitochondrial particle size ( c ) and membrane potential ( d ) were determined using flow cytometry for TMRE in cardiac mitochondria preparations. Results are shown from 4–8 hearts analysed in duplicate. ( e ) H 2 O 2 production with 0.5 mM NADH, complex I-linked substrate, was determined in the absence or presence of 2 μM complex I inhibitor rotenone using Amplex Red ( n =5–8 per group). ( f ) Myocardial high-energy phosphate metabolism under 8γ dobutamine loading was measured biochemically with HPLC ( n =5 per group). ( g ) Maximum dP/dt was examined using cardiac catheterization with graded a dobutamine infusion ( n =5 per group). ( h ) Photographs showing heart sections after SA-β-gal staining; original magnification, × 200; scale bar, 40 μm. SA-β-gal-positive cells were quantified ( n =4 per group). Five images per mouse were taken on brightfield and DAPI staining was used to count the total cell number per section. HT indicates heterozygous; DHT double heterozygous. Data are shown as the means±s.d. * P <0.05; ** P <0.01; *** P <0.001 (two-tailed unpaired Student’s t -test). Full size image Parkin overexpression ameliorates cardiac aging The sustained function of Parkin maintained mitochondrial integrity and cardiac functional reserve in p53 +/− aged littermates. To genetically strengthen the role of mitophagy in the process of aging in vivo , we also generated transgenic mice overexpressing Parkin in cardiomyocytes ( Supplementary Fig. S14a,b ) and monitored phenotypic alterations in cardiac aging. Parkin overexpressing aged hearts exhibited more mitochondria incorporated into autophagosomes, accompanied by less abnormal mitochondria, as compared with age-matched WT hearts ( Fig. 7a–c ). Parkin transgenic mice were resistant to age-dependent mitochondrial alterations accompanied by decreased O 2 consumption ( Fig. 7d ) and an increased level of ROS generation ( Fig. 7f ). Maintained mitochondrial integrity was associated with not only preserved cardiac functional reserve ( Fig. 7g ), but also the attenuation of aging biomarkers including SA-β-gal activity and the expression of cell cycle inhibitors and proinflammatory cytokines ( Fig. 7h–j ). Mitochondrial compromise was closely involved in not only functional decline but also concomitant aging-related alterations. 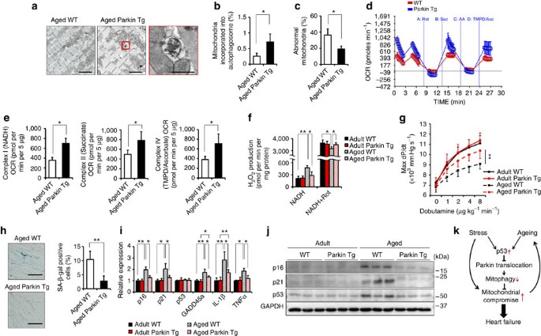Figure 7: Parkin transgenic mice are resistant to cardiac aging. (a) Representative electron micrographs of the heats of 20-month-old aged mice; original magnification × 5,000; scale bar, 2 μm. The magnified photograph shows an autophagic vacuole containing mitochondria; original magnification, × 12,000; scale bar, 500 nm. (b,c) Mitochondria incorporated into an autophagic vacuole (b) and abnormal mitochondria (c) were quantified blindly from 8–10 images from different fields (original magnification × 5,000) (n=3 per group). (d,e) The sequential state III oxygen consumption rate of heart isolated mitochondria was assessed using the Seahorse XF24 Analyser. With the initial presence of 5 μg mitochondria per well, 0.5 mM NADH and 4 μM FCCP, injections were performed as follows: port A, 50 μl of 20 μM rotenone (2 μM final); port B, 55 μl of 100 mM succinate (10 mM final); port C, 60 μl of 40 μM antimycin A (4 μM final); port D, 65 μl of 100 mM ascorbate plus 1 mM TMPD (10 μM and 100 μM final, respectively). Representative results of aged littermates are shown (d) and oxygen consumption by each complex was calculated from four independent experiments, five replicates per sample, and four samples per experiment (n=8 per group,e). (f) NADH-driven H2O2production was determined using Amplex Red. Results are shown from five hearts analysed in duplicate. (g) Maximum dP/dt was examined using cardiac catheterization with graded dobutamine infusion in WT and Parkin Tg aged littermates (n=8 per group). (h) Photographs showing heart sections after SA-β-gal staining; original magnification, × 200; scale bar, 40 μm. SA-β-gal-positive cells were quantified (n=4 per group). Five images per mouse were taken on brightfield and DAPI staining was used to count the total cell number per section. (i) Real-time PCR assessing the expression of cell cycle inhibitors and proinflammatory cytokines (n=8 per group). (j) Representative immunoblots assessing the expression of cell cycle inhibitors are shown; Data are shown as the means±s.d. *P<0.05; **P<0.01 (two-tailed unpaired Student’st-test). (k) Proposed model for mitochondrial compromise in heart failure. Figure 7: Parkin transgenic mice are resistant to cardiac aging. ( a ) Representative electron micrographs of the heats of 20-month-old aged mice; original magnification × 5,000; scale bar, 2 μm. The magnified photograph shows an autophagic vacuole containing mitochondria; original magnification, × 12,000; scale bar, 500 nm. ( b , c ) Mitochondria incorporated into an autophagic vacuole ( b ) and abnormal mitochondria ( c ) were quantified blindly from 8–10 images from different fields (original magnification × 5,000) ( n =3 per group). ( d , e ) The sequential state III oxygen consumption rate of heart isolated mitochondria was assessed using the Seahorse XF24 Analyser. With the initial presence of 5 μg mitochondria per well, 0.5 mM NADH and 4 μM FCCP, injections were performed as follows: port A, 50 μl of 20 μM rotenone (2 μM final); port B, 55 μl of 100 mM succinate (10 mM final); port C, 60 μl of 40 μM antimycin A (4 μM final); port D, 65 μl of 100 mM ascorbate plus 1 mM TMPD (10 μM and 100 μM final, respectively). Representative results of aged littermates are shown ( d ) and oxygen consumption by each complex was calculated from four independent experiments, five replicates per sample, and four samples per experiment ( n =8 per group, e ). ( f ) NADH-driven H 2 O 2 production was determined using Amplex Red. Results are shown from five hearts analysed in duplicate. ( g ) Maximum dP/dt was examined using cardiac catheterization with graded dobutamine infusion in WT and Parkin Tg aged littermates ( n =8 per group). ( h ) Photographs showing heart sections after SA-β-gal staining; original magnification, × 200; scale bar, 40 μm. SA-β-gal-positive cells were quantified ( n =4 per group). Five images per mouse were taken on brightfield and DAPI staining was used to count the total cell number per section. ( i ) Real-time PCR assessing the expression of cell cycle inhibitors and proinflammatory cytokines ( n =8 per group). ( j ) Representative immunoblots assessing the expression of cell cycle inhibitors are shown; Data are shown as the means±s.d. * P <0.05; ** P <0.01 (two-tailed unpaired Student’s t -test). ( k ) Proposed model for mitochondrial compromise in heart failure. Full size image Cardiac mitochondria are the principal integrators of energy production, ROS generation, multiple cell death and signalling pathways in the constantly contracting heart. Accumulating evidence has convincingly demonstrated that structural and functional changes in these multifaceted organelles are implicated in heart failure, myocardial ischaemia and aging [28] . Recently, it became clear that individual mitochondria do not exist as a permanently static organelle, as was originally believed, but instead form a dynamic network within which mitochondria regularly exchange contents by fusion and fission processes. It is now thought that dysfunctional mitochondria are separated from the network by fission and consequently eliminated by macroautophagy to maintain mitochondrial integrity [7] , [29] , and recent experimental results indicate that an impaired dynamic nature and autophagic degradation could be instrumental in aging and heart failure [30] , [31] . Here, we declare for the first time that the process of mitochondrial autophagy is disturbed in aged hearts and senescent cells as well as DOX-treated hearts and cells. A novel protein–protein interaction between cytosolic p53 and Parkin impairs removal of damaged mitochondria by blocking Parkin mitochondrial translocation, which may provide a mechanistic explanation for the observed age-dependent compromise of mitochondrial integrity and functional decline of the heart. In this study, we performed in vivo analysis using global p53 −/− mice that confine to use of heterozygous mice in aged mice studies for its tumorigenesis. Conditional p53 −/− mice in the heart might lead to additional important insights and further support of our conclusions. Contribution of p53 to cellular senescence and the limitation of the proliferative capacity of stem cells [32] may underlay the functional decline of highly proliferative organs. p53 is also involved in aging of more quiescent tissues through the control of inflammatory response [33] and mitochondrial function via downregulation of PGC1 (ref. 34 ). The direct molecular link between p53 activation and Parkin-mediated mitophagy deficiency establishes an additional mechanism of mitochondriopathy which contributes to aging-related alterations including functional multi-system declines and inflammatory states in the context of aging process. The importance of cytosolic p53 in regulating mitophagy was observed in this study. The most-studied function of p53 is its role as a transcription factor that can activate transcription of an ever-increasing number of target genes, whereas p53 also operates at cytosol to modulate cell death and autophagy [35] , [36] , [37] . Genotoxic stress provokes p53 accumulation in both the nucleus and cytosol and endogenous cytosolic p53 can directly activate Bax and thereby induce apoptosis [35] . p53 also functions as an endogenous repressor of autophagy through a cytosolic effect. Some ER stressors and starvation cause the cytoplasmic translocation and subsequent degradation of p53 to induce autophagy [36] . We suggest an additional function of cytosolic p53 in that it inhibits mitophagy by prohibiting Parkin to translocate from cytosol to mitochondria. Moreover, this repressive effect on mitophagy is thought to be independent of the inhibitory influence on bulk autophagy, because p53-mediated effect on mitochondrial quality was abolished by Parkin deletion and the involvement of ER was supposed in cytosolic p53-regulated bulk autophagy [36] , inconsistent with our study. p53 exerts different effects on mitochondrial function according to its expression level. p53 has a short half-life and is maintained at low levels by a continuous ubiquitin proteasome system in non-stressed conditions. At physical levels, p53 is required to maintain the normal transcription of genes associated with oxidative phosphorylation and the mtDNA copy number, including cytochrome c oxidase assembly gene SCO2 (ref. 26 ), mitochondrial transcription factor Tfam [38] and ribonucleotide reductase subunit p53R2 (ref. 39 ). Maximum exercise capacity was shown to be impaired in p53 −/− mice. In contrast, hyper-physiological levels of p53 had the opposite effect on mitochondrial integrity. A recent paper, reporting on telomerase-deficient mice, showed that telomere dysfunction induced a profound p53-dependent repression of the master regulators of mitochondrial biogenesis and respiration, PGC-1α and PGC-1β, which led to a bioenergetic compromise due to impaired oxidative phosphorylation and ATP generation [34] . Our results present another mechanism to promote mitochondrial compromise in the context of aging or DOX-mediated cardiac dysfunction. Similar bilateral behaviours are observed in regulating cellular ROS generation. Activated p53 exerts pro-oxidant activities, whereas basal levels of p53 have a vital function in containing ROS at nontoxic levels through the transactivation of antioxidant genes [40] . Unlike a telomere dysfunction model, the expression of PGC-1α and PGC-1β did not differ with age or p53 genotype in our setting of biological aging and DOX treatment ( Supplementary Fig. S6a,b ). p53 orchestrates the transcription of numerous genes and in many cases, the selective transactivation of certain p53 target genes is achieved in tissue-specific and stress-specific manners. Parkin, E3 ubiquitin ligase, was identified as the gene responsible for autosomal recessive juvenile Parkinsonism (AR-JP) in 1998 (ref. 41 ), and its pathogenicity was found in 2008 (ref. 8 ). Today, the role of Parkin is widely understood in association with other proteins implicated in AR-JP and mitochondrial dynamics. Mitochondria can divide asymmetrically into functional progeny, which can reintegrate the mitochondrial network by fusion, and dysfunctional organelles with low membrane potential, which are specifically destined for mitophagy [9] . In addition to neurodegenerative diseases, Parkin-mediated mitophagy was also shown to contribute to cardiac pathophysiology [42] . Previous studies investigated whether Parkin mutations associated with familial AR-JP were defective in supporting mitophagy. Mutations in the RING2 domain abolished E3 activity of Parkin and other mutations in the RING0 domain were important for the redistribution of Parkin to the damaged mitochondria [43] , consistent with our findings in which cytosolic p53 interacted with the RING0 domain to disturb Parkin translocation. RING0-mediated substrate interactions have been observed in several studies with the K161N mutation [44] , [45] . Among these proteins, BAG5 (bcl-2-associated athanogene 5), a BAG family member, directly interacted with Parkin residues 77–217 (including RING0) in combination with chaperone Hsp70. Within this complex, BAG5 inhibited both Parkin E3 ubiquitin ligase activity and the Hsp70-mediated refolding of misfolded proteins [46] . Further investigations are required to clarify the involvement of BAG5 in the interaction between p53 and Parkin. Recent publications have demonstrated the transcriptional interaction between Parkin and p53. Parkin has been identified as a p53 target gene that decreases glycolysis and increases mitochondrial respiration in association with tumour suppression via a poorly characterized mechanism [47] . In addition, Parkin was shown to be a transcriptional repressor of p53 in neural cells in the context of AR-JP pathology [48] . These interactions were not observed in hearts and cardiac myocytes examined in this study. The mRNA expression of Parkin did not differ in the heart with age or p53 genotype ( Supplementary Fig. S6a,b ). Parkin protein expression also did not change under p53-activating stress ( Fig. 3b ). Furthermore, Parkin overexpression in the heart and cardiac myocytes did not exhibit any effects on p53 transcription ( Fig. 7i , Supplementary Fig. S4b ). Given these results, it is fair to conclude that previously reported p53-Parkin transcriptional regulations did not affect the inhibitory protein interaction of p53 with Parkin, at least in the heart. We observed the beneficial effects of Parkin overexpression on mitochondrial bioenergetics in aged cardiomyocytes. Although Parkin-mediated PGC-1α expression reported by Shin et al . [49] could be a candidate mechanism of mitochondrial protection, we did not observe significant upregulation of PGC-1α in Parkin overexpressing hearts and myocytes ( Supplementary Figs S14a,S4b ). This regulation was only demonstrated in the ventral midbrain, indicating an intensive region specific manner. Moreover, they mentioned only the repressive effects of the loss-of-function of Parkin, not the benefits of gain-of-function. In summary, our present study provides molecular understandings of mitochondrial deficiency in heart failure. Cytosolic p53 inhibits Parkin-mediated mitophagy and provokes mitochondrial compromise involved in aging-related and DOX-mediated decreases in cardiac contractility. We provide a novel concept as illustrated in Fig. 7k ; the cascade of p53 activation and Parkin-mediated mitophagy deficiency accelerates a vicious cycle of mitochondrial compromise and aging. Together with the classical cellular outcomes of p53 activation such as senescence and apoptosis, this vicious cycle contributes to age-dependent declines of organismal fitness and performance. The activation of mitophagy could be a novel target to alleviate heart diseases that are especially caused by aging or mitochondrial dysfunction. Mice experiments All animal studies were approved by the Bioethics Committee of Kyoto Prefectural University of Medicine. p53-deficient mice (C57BL/6J background), Parkin-deficient mice [50] (C57BL/6J background) and p21-deficient mice (C57BL/6J background) were obtained from the Jackson Laboratory. p53-deficient mice and Parkin-deficient mice were mated to generate double heterozygotes. Double heterozygous pairing produced p53 +/+ Parkin +/+ , p53 −/− Parkin +/+ , p53 +/+ Parkin −/− and p53 −/− Parkin −/− mice. Male mice were used in this study. As the pathological aging model, these mice were administrated DOX in five equal intraperitoneal injections (each containing 2.5 mg kg −1 ) over a period of 2 weeks, with a total cumulative dosage of 12.5 mg kg −1 at 10 weeks of age, and were killed at 18 weeks of age. GFP-LC3 transgenic mice (strain GFP-LC3 no. 53, C57BL/6J background) were purchased from RIKEN BioResource Center. We generated a heart-specific Parkin transgenic mice (C57BL/6J background). The Parkin transcript was amplified from mouse heart total RNA using Parkin-specific primers. Parkin cDNA was cloned into plasmid Clone 26 provided by Dr Jeffrey Robbins (University of Cincinnati) to recruit the 5.4-kb mouse α-myosin heavy chain promoter [51] . The transgenic construct was released from the prokaryotic backbone and injected into the pronucleus of C57BL/6J embryos at the one-cell stage (UNITECH, Japan). Transgenic mice were maintained by sibling mating and used as hemizygotes. Cell culture HL-1 cardiomyocytes were obtained from Dr W.C. Claycomb (Louisiana State University) [52] . Cells were cultured on a gelatin (0.02% (wt/vol))/fibronectin (10 μg ml −1 ) matrix and were maintained in Claycomb medium (JRH Biosciences) supplemented with 10% fetal bovine serum (FBS), 2 mM glutamine, 0.1 mM norepinephrine, 100 U ml −1 penicillin and 100 μg ml −1 streptomycin. Three different p53 genotypes of HCT116 human colon cancer cell lines: WT (+/+) heterozygous (+/−) and homozygous (−/−) were generous gifts from Dr Bert Vogelstein (Johns Hopkins University) [53] . Cells were grown in McCoy’s 5A medium supplemented with 10% FBS containing 100 U ml −1 penicillin and 100 μg ml −1 streptomycin. Mouse embryonic fibroblasts (MEFs) were prepared from C57/BL6J mouse embryos at embryonic day 13.5 and cultured in DMEM plus 10% FBS containing 100 U ml −1 penicillin and 100 μg ml −1 streptomycin. MEFs at passage 9 became flattened large cells positive for senescence-associated β-galactosidase (SA-β-Gal), and did not show an increase of cell number and remained subconfluent for 2 weeks. MEFs at passage 3 and 9 were used as young and senescent MEFs, respectively. Plasmids and RNA interference YFP-Parkin and GFP-p53(NES−) were purchased from Addgene. p53 WT and p53 ER were gifts from Dr Moll UM (Stony Brook University) [54] . p53 WT and mutants were reinserted into Bam HI site of pcDNA3.1 (Invitrogen) to remove GFP using In-Fusion HD Cloning Kits (Clontech). p53(NLS−) and transcript variants were cloned using the p53 WT vector as a template and inserted into the Bam HI site of pcDNA3.1 (Invitrogen). Plasmids were transfected using Lipofectamine 2000 (Invitrogen) according to the product protocol. Mouse p53, p21 and p16-specific siRNA duplexes were purchased from Invitrogen. siRNAs were transiently transfected using Lipofectamine RNAiMAX (Invitrogen) according to the product protocol. Sequences of siRNA are provided in Supplementary Table S1 . Recombinant retrovirus construction H-RAS V12 retroviral vector was purchased from Addgene and reinserted into the site of Bgl II of pMSCV-puro retroviral construct using In-Fusion HD Cloning Kits (Clontech). Mouse p53, p21, p16, Rb were cloned and inserted into the site of Bgl II of pMSCV-puro retroviral construct. Briefly, HEK293T cells were transfected with plasmids expressing retroviral proteins using Lipofectamine 2000 (Invitrogen). At 48 h after transfection, supernatants containing the retroviral particles were collected and frozen at −80 °C until use. Cells were infected with diluted supernatant in the presence of 10 μg ml −1 Polybrene for 6 h, and 24 h after infection, selected for at least 8 days in the presence of 0.75 μg ml −1 puromycin. Recombinant adenovirus construction The cDNAs encoding mouse Parkin, and LacZ were inserted into a pAxCAwtit cosmid vector in an adenovirus expression vector kit (Dual Version; Takara Bio Inc.) according to the product protocol. Adenovirus expressing GFP-LC3 was a kind gift from Dr T. Yoshimori (Osaka University). Cells were infected with adenovirus that was diluted in the culture medium at a multiplicity of infection (MOI) of 5–50 and incubated at 37 °C for 1 h. Cardiac hemodynamics in vivo Mice were anesthetized with 2,2,2-tribromoethanol (0.25 mg g −1 of body weight; Aldrich), subsequently anesthetized with isoflurane (1.5% (vol/vol) in O 2 ) and placed on a 36.5 °C table. Both vagal nerves were cut, and the right jugular vein was cannulated with stretched polythene tubing for intravenous infusions. Through the right carotid artery, a 1.2 French Millar type catheter-tip micromanometer catheter (Scisense) was inserted via a small incision, and the tip was manipulated across the aortic valve into the LV. Following the stabilization of hemodynamic conditions, dobutamine was given intravenously by an infusion pump (KDS100; KD Scientific), at a rate of 1, 2, 4 and 8 μg kg −1 min −1 . LV pressure signals of 10 to 20 beats were averaged and analysed with PowerLab software (Chart 5. AD Instruments). Mitochondrial isolation Mouse hearts were rapidly minced in ice cold MSE buffer (220 mM mannitol, 70 mM sucrose, 2 mM EGTA, 5 mM MOPS (pH 7.4), 2 mM taurine and 0.2% BSA). Heart tissue was homogenized in MSE buffer with a polytron type tissue grinder at 11,000 r.p.m. for 2.5 s followed by two quick strokes at 500 r.p.m. with a loose fit Potter-Elvenhjem tissue grinder. The homogenate was centrifuged at 500 g twice for 5 min saving the supernatant. Pellet mitochondria from the supernatant at 3,000 g twice, rinsing the pellet with MSE buffer. The final pellet was rinsed and resuspended in 50 μl incubation medium (220 mM mannitol, 70 mM sucrose, 1 mM EGTA, 5 mM MOPS (pH 7.4), 2 mM taurine, 10 mM MgCl 2 , 5 mM KH 2 PO 4 and 0.2% BSA). Mitochondria were incubated for 15 min on wet ice and protein concentrations were determined with BSA as a standard by a Bradford assay. All work was performed on wet ice. Immunoblot and immunoprecipitation Antibodies used for immunoblotting included mouse anti-p53 (1:1,000, DO-1, Santa Cruz), gout anti-p53 (1:500, C-19, Santa Cruz), mouse anti-p53 (1:1,000, no. 2524, Cell signaling), rabbit anti-Parkin (1:1,000, ab15954, Abcam), mouse anti-Parkin (1:1,000, no. 4211, Cell signaling), guinea-pig anti-p62 (1:1,000, GP62-C, Progen), rabbit anti-PINK1 (1:1,000, BC100-494, Novus), gout anit-GRP75 (1:1,000, sc-13967, Santa Cruz), mouse anti-NDUFA9 (1:2,000, 459100, Invitrogen), rabbit anti-Mfn1 (1:500, 13798-1-AP, Proteintech), rabbit anti-Drp1 (1:500, no. 8570, Cell signaling), mouse anti-ATP synthase α (1:2,000, 459240, Invitrogen), mouse anti-GAPDH (1:2,000, MAB374, Millipore), mouse anti-GST (1:1,000, 011-21891, WAKO), mouse anti-Poly-ubiquitin (1:1,000, FK-2, MBL), gout anti-LDH (1:1,000, ab2101, Abcam), mouse anti-VDAC (1:2,000, 43841A, Invitrogen), mouse anti-Flag (1:2,000, M2, Stratgene), rabbit anti-PGC-1α (1:1,000, 101707, Cayman), mouse anti-GFP (1:1,000, JL8, Living colours), mouse anti-p16 (1:500, sc-1661, Santa Cruz), rabbit anti-p21 (1:500, sc-397, Santa Cruz), mouse anti-H-Ras (1:500, MAB3291, Millipore), mouse anti-Rb (1:500, 554136, BD Pharmingen). HRP-conjugated secondary antibodies were obtained from Amersham Pharmacia and Millipore. PVDF membrane (BioLad) was used for blotting and signals were revealed by ECL prime (GE healthcare). For immunoprecipitation, HL-1 rat neonatal cardiomyocytes were treated in the lysis buffer (50 mM Tris-HCl, 150 mM NaCl, 1% NP-40, 1 mM DTT, 1 mM EGTA, 1 mM Na3VO4, 50 mM NaF, supplemented with mammalian protease inhibitor cocktail: Sigma-Aldrich). Cell lysate (200 μg protein) was subjected to immunoprecipitation with antibodies coupled to magnetic beads (Magnosphere MS300/Carboxyl, JSR) or GFP-Trap coupled to magnetic particles (Chromotek). After the beads were washed, samples were boiled with sample buffer and subjected to immunoblotting. Full-length images of immunoblots are shown in Supplementary Fig. S15 . Immunofluorescence MEFs infected with adenovirus expressing Parkin and GFP-LC3, HL-1 cells transfected with GFP-mParkin or HCT116 cells transfected with YFP-hParkin and various mutant p53 were treated with CCCP. The sample was fixed by 4% paraformaldehyde, permeabilized with methanol/acetone and stained with antibodies. Heart samples of GFP-LC3 Tg mice were prepared as follows. To prevent induction of autophagy during tissue preparation, mice were immediately fixed by perfusion through the left ventricle with 4% paraformaldehyde. Hearts were harvested and further fixed with the same fixative for at least 4 h, followed by treatment with 15% sucrose in PBS for 4 h and then with 30% sucrose solution overnight. Tissue samples were embedded in Tissue-Tek OCT compound (Sakura Finetechnical Co. Ltd) and stored at −80 °C. The samples were sectioned at 7 μm thickness with a cryostat (CM3050 S, Leica), air-dried for 30 min and followed by permeabilization with methanol/acetone and staining with antibodies. We used the following antibodies: rabbit anti-TOM20 (1:200, sc-11415, Santa Cruz), mouse anti-poly-ubiquitin (1:200, FK-2, MBL), mouse anti-p53 (1:200, DO-1, Santa Cruz), gout anti-p53 (1:100, C-19, Santa Cruz), rabbit anti-Calnexin (1:200, no. 2433, Cell signaling), mouse anti-α-sarcomeric actinin (1:200, A7811, Sigma). Samples were mounted using VectaShield with DAPI mounting medium (H-1200; Vector Laboratories), and observed under a fluorescence confocal microscope (LSM510 META, Carl Zeiss). Statistical analysis Data are shown as the mean±s.d. Statistical comparisons were made using the two-tailed unpaired Student’s t -test. A probability value of <0.05 was considered to indicate statistical significance. Statistical analysis was performed using Excel software. How to cite this article: Hoshino, A. et al . Cytosolic p53 inhibits Parkin-mediated mitophagy and promotes mitochondrial dysfunction in the mouse heart. Nat. Commun. 4:2308 doi: 10.1038/ncomms3308 (2013).